The Hedgehog signalling pathway regulates autophagy Autophagy is a highly conserved degradative process that removes damaged or unnecessary proteins and organelles, and recycles cytoplasmic contents during starvation. Autophagy is essential in physiological processes such as embryonic development but how autophagy is regulated by canonical developmental pathways is unclear. Here we show that the Hedgehog signalling pathway inhibits autophagosome synthesis, both in basal and in autophagy-induced conditions. This mechanism is conserved in mammalian cells and in Drosophila , and requires the orthologous transcription factors Gli2 and Ci, respectively. Furthermore, we identify that activation of the Hedgehog pathway reduces PERK levels, concomitant with a decrease in phosphorylation of the translation initiation factor eukaryotic initiation factor 2α, suggesting a novel target of this pathway and providing a possible link between Hedgehog signalling and autophagy. Autophagy is a bulk degradative pathway in which damaged organelles and cytoplasmic proteins are engulfed in double-membrane vesicles called autophagosomes, which then fuse with lysosomes where their contents are degraded. Autophagy occurs at low levels in basal conditions and it can be upregulated by starvation, or with chemicals such as rapamycin or trehalose [1] . Autophagy dysfunction is associated with different human pathologies, including cancer, neurodegeneration or bacterial infection. But autophagy also maintains normal homeostasis by degrading misfolded proteins and organelles, and by releasing nutrients when these are limiting. These aspects are vital during embryonic development, where cells undergo periods of rapid cell growth and enhanced metabolism, differentiation or cell death. There is growing evidence pointing to autophagy as a key factor during embryogenesis. Mice deficient in autophagy genes such as Beclin1 have early embryonic lethality [2] and Atg5-knockout mice die perinatally [3] (reviewed in Cecconi and Levine [4] ). Early embryonic development is controlled by central signalling pathways such as Wnt, Notch or Hedgehog (Hh). Although autophagy has recently been shown to activate the Wnt pathway [5] , the signal transduction pathways regulating autophagy in the developing embryo are unclear. Autophagy seems to be important during neural tube development, as embryos with loss of function of Ambra1 (which positively regulates autophagy) have neural tube defects and early embryonic lethality [6] and Atg5 and Ambra1 are necessary for neurogenesis [7] . Hh signalling is of particular interest because this pathway is responsible for the correct development of the neural tube and induction of ventral neural fate (reviewed in Dessaud [8] ). Most key molecular components of Hh pathway are conserved between mammals and Drosophila , where the pathway was first identified. In both vertebrates and invertebrates, binding of the Hh family of secreted proteins to the transmembrane receptor patched (Ptch) releases catalytically repressed smoothened (Smo) [9] . Ultimately, Smo signalling stabilizes the active form of the Drosophila transcription factor Cubitus interruptus (Ci), that otherwise would be catalytically processed, releasing a repressor form which inhibits the expression of Hh target genes. In mammalian cells, three Ci orthologs, Gli1, Gli2 and Gli3, mediate Hh transcriptional responses. Although Gli1 and Gli2 are responsible for activator functions, the absence of ligand results in Gli3 (and possibly Gli2) processing to a truncated repressor form [10] . Here we describe that Hh signalling impairs autophagy. We have dissected the contribution that different components of this pathway have on autophagy flux in mammalian cells, as well as in Drosophila . Our data suggest that autophagy is regulated by the canonical Hh pathway and that Ci in Drosophila and Gli2 in mammals are key modulators in this response. Activation of Hh signalling impairs autophagy We first treated HeLa cells with an N-terminal recombinant Sonic Hh peptide (N-Shh) and measured LC3-II protein levels [11] . LC3 (microtubule-associated protein 1 light chain 3) is processed post-translationally into cytosolic LC3-I, and upon autophagy induction is converted to its lipidated form, LC3-II, which specifically associates with autophagosome membranes. Therefore, LC3-II levels on western blots reflect autophagosome numbers. LC3-II levels were reduced by N-Shh compared with untreated cells in basal autophagy conditions ( Fig. 1a ). 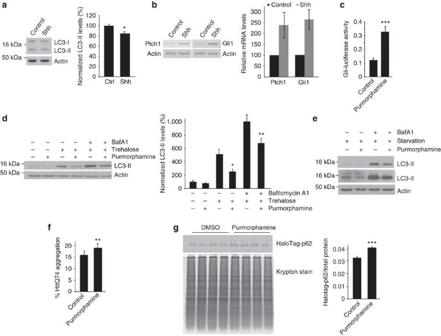Figure 1: Autophagy is inhibited in the presence of Hh agonists. (a,b) HeLa cells were treated with 10 μg ml−1N-Shh peptide for 24 h. (a) Endogenous LC3 was detected by immunoblot in total cell lysates, quantified by densitometric analysis and normalized to actin. Relative levels were expressed in percentage with control cells set to 100 and shown in graph. (b) mRNA was obtained and levels of Ptch1 or Gli1 and actin mRNA were amplified by standard PCR and visualized in agarose gels. Graph shows mRNA levels quantified by densitometric analysis and normalized to actin. (c) 8xGli-luciferase construct was transfected in HeLa cells for 24 h, followed by treatment with 10 μM purmorphamine, or DMSO as a control, for another 24 h. Graph represents the mean value of thefireflyluciferase activity relative toRenillatransfection control. (d) Endogenous LC3-II was detected in cell lysates from cells treated with 10 μM purmorphamine for 24 h, either in the absence or presence of trehalose (100 mM). Where indicated, bafA1 (400 nM) was added for the last 4 h. Quantification by densitometric analysis relative to actin is shown in the graph. (e) Cells were treated with 10 μM purmorphamine for 24 h under starvation conditions, either in the presence of bafA1 or DMSO as a control, and LC3-II and actin levels were detected. (f) HA-HttQ74 construct was transfected into HeLa cells followed by treatment with 10 μM purmorphamine for 24 h. The percentage of transfected cells with aggregates detected by HA immunofluorescence is shown in the graph.P-values were calculated by odds ratio. (g) U20S cells stably expressing HaloTag-p62 were labelled with HaloTag ligand for 15 min and washed out followed by treatment with purmorphamine. After 48 h, cells were lysed, run on a SDS–polyacrylamide gel electrophoresis and fluorescent HaloTag was visualized using a Typhoon 8600 variable mode imager. Fluorescence was normalized to total protein levels, detected on the same gels by Kryton Fluorescence protein stain. A representative gel and its quantitated normalized levels are shown. In all panels, graphs show mean values and error bars represent s.d. from a triplicate experiment representative of at least three independent experiments. Statistical analyses were performed by two-tail Student’st-test unless indicated: ***P<0.001; **P<0.01; *P<0.05. SDS–PAGE, SDS–polyacrylamide gel electrophoresis. Figure 1: Autophagy is inhibited in the presence of Hh agonists. ( a , b ) HeLa cells were treated with 10 μg ml −1 N-Shh peptide for 24 h. ( a ) Endogenous LC3 was detected by immunoblot in total cell lysates, quantified by densitometric analysis and normalized to actin. Relative levels were expressed in percentage with control cells set to 100 and shown in graph. ( b ) mRNA was obtained and levels of Ptch1 or Gli1 and actin mRNA were amplified by standard PCR and visualized in agarose gels. Graph shows mRNA levels quantified by densitometric analysis and normalized to actin. ( c ) 8xGli-luciferase construct was transfected in HeLa cells for 24 h, followed by treatment with 10 μM purmorphamine, or DMSO as a control, for another 24 h. Graph represents the mean value of the firefly luciferase activity relative to Renilla transfection control. ( d ) Endogenous LC3-II was detected in cell lysates from cells treated with 10 μM purmorphamine for 24 h, either in the absence or presence of trehalose (100 mM). Where indicated, bafA1 (400 nM) was added for the last 4 h. Quantification by densitometric analysis relative to actin is shown in the graph. ( e ) Cells were treated with 10 μM purmorphamine for 24 h under starvation conditions, either in the presence of bafA1 or DMSO as a control, and LC3-II and actin levels were detected. ( f ) HA-HttQ74 construct was transfected into HeLa cells followed by treatment with 10 μM purmorphamine for 24 h. The percentage of transfected cells with aggregates detected by HA immunofluorescence is shown in the graph. P -values were calculated by odds ratio. ( g ) U20S cells stably expressing HaloTag-p62 were labelled with HaloTag ligand for 15 min and washed out followed by treatment with purmorphamine. After 48 h, cells were lysed, run on a SDS–polyacrylamide gel electrophoresis and fluorescent HaloTag was visualized using a Typhoon 8600 variable mode imager. Fluorescence was normalized to total protein levels, detected on the same gels by Kryton Fluorescence protein stain. A representative gel and its quantitated normalized levels are shown. In all panels, graphs show mean values and error bars represent s.d. from a triplicate experiment representative of at least three independent experiments. Statistical analyses were performed by two-tail Student’s t -test unless indicated: *** P <0.001; ** P <0.01; * P <0.05. SDS–PAGE, SDS–polyacrylamide gel electrophoresis. Full size image We performed this and further experiments in HeLa cells, which allow efficient short interfering RNA (siRNA) silencing and DNA transfection. We confirmed efficient Hh pathway activation in these cells by showing that N-Shh increases mRNA levels of Ptch1 and Gli1, known transcriptional targets of this pathway [12] , [13] ( Fig. 1b ). We also verified that purmorphamine [14] , another Hh agonist, activated Hh signalling in our cells using a well-established 8xGli-luciferase reporter [15] ( Fig. 1c ). Similar to N-Shh, purmorphamine reduced steady-state LC3-II levels ( Fig. 1d ). Purmorphamine also reduced LC3-II in conditions in which autophagy is induced by starvation or rapamycin ( Fig. 1e and Supplementary Fig. S1A ). Starvation and rapamycin stimulate autophagy through mechanisms involving mammalian target of rapamycin (mTOR) kinase inactivation [16] , and it has been reported that mTOR [17] and the phosphoinositide 3-kinase/AKT pathway [18] , which acts upstream of mTOR, regulate Hh signalling. To avoid the possible complexities of cross-talk of this pathway with Hh, we used trehalose to induce autophagy independently of mTOR activity [19] . As shown in Fig. 1d , trehalose greatly increases LC3-II levels. In these conditions, the addition of 10 μM purmorphamine counteracted trehalose induction of autophagy, indicating that purmorphamine can reduce both basal and induced autophagy. A decrease in LC3-II could result from inhibition of autophagosome formation or enhanced autophagosome clearance. Measurement of LC3-II levels in the presence of bafilomycin A1 (bafA1), which blocks autophagosome-lysosome fusion, allows deconvolution of these two possibilities [20] . As purmorphamine decreased LC3-II in the presence of bafA1 ( Fig. 1d ), the Hh pathway affects autophagosome synthesis rather than autophagosome degradation. To further confirm these data, we assessed whether Hh activation influenced autophagy substrate accumulation. Cells expressing HA-tagged huntingtin exon 1 with 74 polyglutamine (HA-HttQ74) form intracellular aggregates and the percentage of cells with aggregates correlates with protein concentration [21] . As HttQ74 clearance is highly dependent on autophagy, the proportion of cells with visible aggregates correlates inversely with autophagic activity (if other factors are kept constant) [16] . Consistent with a reduction in LC3-II levels, purmorphamine increased the percentage of cells with HttQ74 aggregates ( Fig. 1f ). We also examined the soluble autophagy substrate, p62/SQSTM1 ( [22] ), by generating U2OS-stable cell lines expressing HaloTag-p62, which were incubated with a fluorescent HaloTag fluorescent ligand that binds covalently and irreversibly to the HaloTag protein. This allows a pool of the protein to be fluorescently labelled and its clearance to be followed over time after ligand binding, as described recently [23] . Autophagy activation by rapamycin or trehalose decreases HaloTag-p62 levels, whereas bafA1 delays its clearance ( Supplementary Fig. S1B ). Purmorphamine slowed the clearance of HaloTag-p62 ( Fig. 1g ) consistent with a decrease in protein clearance and impaired autophagy by Hh activation. Hh regulates autophagy through Ptch1 and Ptch2 In the absence of Hh ligands, two transmembrane receptors, Ptch1 and Ptch2, inhibit another transmembrane protein, Smo. Shh binds to Ptch1/Ptch2 and prevents them from inhibiting Smo, thereby activating the pathway. Ptch1 or Ptch2 overexpression ( Supplementary Fig. S2A ) (which inhibits Hh signalling), increased LC3-II levels in the absence and presence of bafA1 ( Fig. 2a ) and decreased the percentages of HeLa cells and wild-type mouse embryonic fibroblasts (MEFs) with HttQ74 aggregates ( Fig. 2b ). This effect was abolished in autophagy-incompetent, Atg5-deficient (MEFs) [24] ( Fig. 2c ), suggesting that Ptch1/Ptch2 modulate aggregation in an autophagy-dependent manner. 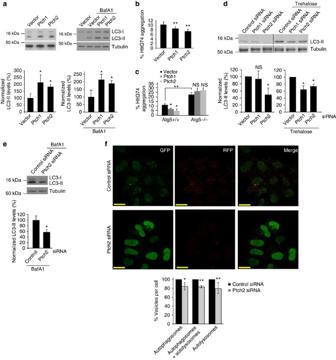Figure 2: Ptch1 and Ptch2 receptors regulate autophagosome synthesis. (a) HeLa cells were transiently transfected with pcDNA (vector), Ptch1 or Ptch2 constructs for 48 h. Where indicated, cells were treated with bafA1 for the last 4 h. LC3-II levels were detected by western blotting and levels were quantified by densitometric analysis relative to tubulin and shown in graph. (b) HeLa were transfected with Ptch1 or Ptch2 together with HA-HttQ74 and the percentage of transfected cells with aggregates was assessed by HA immunofluorescence.P-values were calculated by odds ratio. (c) Atg5+/+ or Atg5−/− MEFs were transfected with GFP-HttQ74 for 48 h, cells were fixed and the percentage of transfected cells with aggregates was scored by direct fluorescence. (d,e) Endogenous LC3-II levels were detected in HeLa cells transfected with control, Ptch1 or Ptch2 siRNA and either left untreated or treated with 100 mM trehalose in the last 24 h (d) or 400 nM bafA1 for 4 h (e). Quantification and statistical analysis is shown in graphs. (f) siRNA-targeting Ptch2 was transfected into HeLa cells stably expressing mRFP-GFP-LC3 and representative confocal microscopy images are shown. Scale bars represent 26 μm. Percentage of GFP-positive vesicles (autophagosomes), RFP-positive vesicles (total number of vesicles) or percentage of autolysosomes (calculated by subtracting numbers of GFP from RFP vesicles), quantified using a Cellomics array scan, was calculated relative to control siRNA-transfected cells. Although an increase in autophagosome biogenesis generally increases both the number of GFP+ vesicles and the number of GFP-/RFP+ vesicles as a result of an enhanced autophagy flux, defects in autophagosome degradation, such as in bafA1-treated cells, increase GFP+ vesicles but not GFP−/RFP+ structures, as GFP remains intact. Graph shows the mean value obtained from four independent experiments in triplicate and with control conditions set to 100. In all panels, unless indicated, graphs show mean values and error bars represent s.d. from a triplicate experiment representative of at least three independent experiments. Statistical analyses were performed by two-tail Student’st-test: **P<0.01; *P<0.05; NS, not significant. Figure 2: Ptch1 and Ptch2 receptors regulate autophagosome synthesis. ( a ) HeLa cells were transiently transfected with pcDNA (vector), Ptch1 or Ptch2 constructs for 48 h. Where indicated, cells were treated with bafA1 for the last 4 h. LC3-II levels were detected by western blotting and levels were quantified by densitometric analysis relative to tubulin and shown in graph. ( b ) HeLa were transfected with Ptch1 or Ptch2 together with HA-HttQ74 and the percentage of transfected cells with aggregates was assessed by HA immunofluorescence. P -values were calculated by odds ratio. ( c ) Atg5+/+ or Atg5−/− MEFs were transfected with GFP-HttQ74 for 48 h, cells were fixed and the percentage of transfected cells with aggregates was scored by direct fluorescence. ( d , e ) Endogenous LC3-II levels were detected in HeLa cells transfected with control, Ptch1 or Ptch2 siRNA and either left untreated or treated with 100 mM trehalose in the last 24 h ( d ) or 400 nM bafA1 for 4 h ( e ). Quantification and statistical analysis is shown in graphs. ( f ) siRNA-targeting Ptch2 was transfected into HeLa cells stably expressing mRFP-GFP-LC3 and representative confocal microscopy images are shown. Scale bars represent 26 μm. Percentage of GFP-positive vesicles (autophagosomes), RFP-positive vesicles (total number of vesicles) or percentage of autolysosomes (calculated by subtracting numbers of GFP from RFP vesicles), quantified using a Cellomics array scan, was calculated relative to control siRNA-transfected cells. Although an increase in autophagosome biogenesis generally increases both the number of GFP+ vesicles and the number of GFP-/RFP+ vesicles as a result of an enhanced autophagy flux, defects in autophagosome degradation, such as in bafA1-treated cells, increase GFP+ vesicles but not GFP−/RFP+ structures, as GFP remains intact. Graph shows the mean value obtained from four independent experiments in triplicate and with control conditions set to 100. In all panels, unless indicated, graphs show mean values and error bars represent s.d. from a triplicate experiment representative of at least three independent experiments. Statistical analyses were performed by two-tail Student’s t -test: ** P <0.01; * P <0.05; NS, not significant. Full size image To confirm the roles of endogenous Ptch1 and Ptch2, we silenced the expression of each receptor with siRNAs, either in basal conditions or in the presence of trehalose. Owing to the lack of antibodies that efficiently recognize endogenous Ptch1 and Ptch2, we confirmed the efficiency of these siRNAs in cells overexpressing Ptch1 or Ptch2 ( Supplementary Fig. S2A ). As expected, knockdown of Ptch1 or Ptch2 reduced LC3-II levels when autophagy was upregulated by trehalose treatment ( Fig. 2d ). In uninduced conditions, however, only Ptch2 siRNA caused a significant decrease of LC3-II. These differences could be explained by Ptch1 siRNA having a smaller effect on Hh signalling compared with Ptch2 knockdown, evaluated using the Gli-reporter assay ( Supplementary Fig. S2B ). Consequently, we used Ptch2 siRNA to further explore the role of Hh on autophagy flux. Different approaches can help to determine whether changes in LC3-II correspond to variations in autophagosome synthesis or in the maturation process. Ptch2 siRNA reduced LC3-II levels in cells treated with bafA1 ( Fig. 2e ). Another approach allows one to differentiate between the LC3 located on either autophagosomes or autolysosomes by using LC3 tagged with mRFP and green fluorescent protein (GFP) in tandem (mRFP-GFP-LC3). Owing to the different pKa values of these fluorescent proteins (GFP pKa is around 6, whereas red fluorescent protein (RFP) pKa is lower than 4.5), their stability differs in the different compartments. In autophagosomes, both GFP and RFP are stable, however, after fusion with the lysosome and acidification, the GFP signal is lost and only RFP is detected [25] . We confirmed that the percentage of only autophagosomes (GFP+ vesicles), autophagosomes plus autolysosomes (total RFP+ vesicles) and the number of autolysosomes (vesicles RFP+ but GFP−) was lower in Ptch2-knockdown cells relative to cells treated with siRNA control ( Fig. 2f ), confirming that Ptch2 siRNA impairs autophagosome synthesis without affecting the fusion process. To further explore the mechanism by which Hh inhibits autophagy, we assessed whether this effect depends on mTOR. Activation of mTOR kinase activity can be monitored by the phosphorylation state of substrates, like the initiation factor 4E-binding protein or p70 ribosomal S6 protein kinase (p70S6K). Although rapamycin reduced S6 protein phosphorylation (a substrate of p70S6K) relative to total protein levels and changed the phosphorylation pattern of 4E-binding protein, no changes were observed upon activation of Hh by Ptch2 siRNA treatment or inhibiting the pathway by overexpressing Ptch1 ( Supplementary Fig. S2C ). These data indicate that suppression of autophagy by Hh is not mediated by mTOR. Hh-regulated autophagy requires Smo Downstream of Ptch1 and Ptch2, the transmembrane protein Smo transmits the Hh response and, consistent with our hypothesis, it should exert a negative role on autophagy. In line with our previous experiments, we transfected cultured cells with a wild-type form of Smo (Smo-myc) or a constitutively active version of the protein carrying an oncogenic mutation (W539L; SmoA1-Myc) [26] ( Supplementary Fig. S3A ). LC3-II levels were decreased in trehalose-induced autophagy conditions in the presence of SmoA1 ( Supplementary Fig. S3B ). Conversely, treatment with Smo siRNA decreased HttQ74 accumulation compared with control siRNA-treated cells ( Fig. 3a ). Similarly, Smo siRNA transfected in cells expressing mRFP-GFP-LC3 increased the number of autophagosomes as well as the number of autolysosomal/RFP-only-positive vesicles ( Fig. 3b ), suggesting that Hh signalling requires Smo to modulate autophagosome synthesis. Similar to Ptch1 and Ptch2, due to the lack of antibodies recognizing endogenous Smo, knockdown efficiency was confirmed after treating cells expressing Smo-GFP with Smo siRNA ( Supplementary Fig. S3C ). 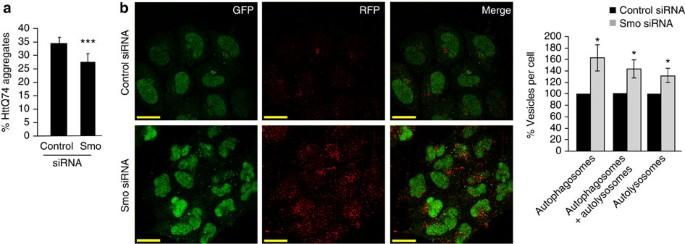Figure 3: Smoothened knockdown increases autophagy. (a) Smo siRNA-treated cells were transfected with HA-HttQ74 for the last 24 h and the percentage of transfected cells with aggregates scored in HA-positive cells by immunofluorescence. Graphs show mean values and error bars represent s.d. of a representative experiment performed in triplicate.P-values were calculated by odds ratio. (b) siRNA-targeting Smo was transfected into HeLa cells stably expressing mRFP-GFP-LC3. Representative confocal microscopy images are shown. Bars represent 26 μm. The number of vesicles was analyzed in a Cellomics array scan and percentage was calculated relative to control siRNA-transfected cells. Statistical tests were performed on data from three independent experiments in triplicate. *P<0.05; ***P<0.001. Figure 3: Smoothened knockdown increases autophagy. ( a ) Smo siRNA-treated cells were transfected with HA-HttQ74 for the last 24 h and the percentage of transfected cells with aggregates scored in HA-positive cells by immunofluorescence. Graphs show mean values and error bars represent s.d. of a representative experiment performed in triplicate. P -values were calculated by odds ratio. ( b ) siRNA-targeting Smo was transfected into HeLa cells stably expressing mRFP-GFP-LC3. Representative confocal microscopy images are shown. Bars represent 26 μm. The number of vesicles was analyzed in a Cellomics array scan and percentage was calculated relative to control siRNA-transfected cells. Statistical tests were performed on data from three independent experiments in triplicate. * P <0.05; *** P <0.001. Full size image Downregulation of autophagy by Hh is Gli2 dependent We next tested the roles of the different Gli transcription factors in autophagy regulation by Hh. Both Gli1 and Gli2 act as transcriptional activators in the presence of Shh [27] . Despite their similarity, loss of Gli2 is embryonically lethal [28] , whereas Gli1 is not essential for normal development [29] . In the absence of ligand, Gli3 is proteolytically processed and functions as a transcriptional repressor [30] . Studying the role of the different Gli transcription factors through overexpression or knockdown experiments is not easy, due to possible redundant or opposite effects that would unmask the real contribution of each factor to autophagy. Therefore, we decided to characterize their effects using embryonic fibroblasts from Gli-knockout mice [31] . To eliminate the clonal differences between the different MEF lines, we examined the capacity of each knockout cell line to respond to the treatment with purmorphamine. As expected, purmorphamine decreased LC3-II in wild-type MEFs treated with trehalose ( Fig. 4a ). Cells deficient for Gli1 or Gli3 were able to respond to purmorphamine which impaired autophagy in the same way we observed in wild-type MEFs. However, in the absence of Gli2, purmorphamine was not able to reduce LC3-II levels. These results indicate that Hh signalling requires intact Gli2 to regulate autophagy upon activation of Hh signalling. 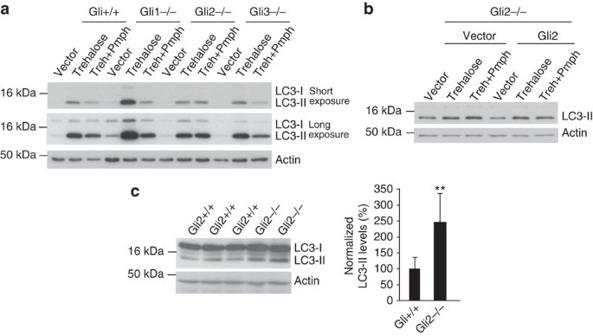Figure 4: Hh regulation of autophagy is Gli2 dependent. (a) Wild-type Gli+/+ or Gli1−/−, Gli2−/− and Gli3−/− MEFs were treated with 100 mM trehalose alone or in combination with 10 μM of Pmph for 24 h, or left untreated. Total cell lysates were subjected to immunoblot with anti-LC3 and anti–actin antibodies. (b) Gli2−/− MEFs were transfected for 48 h with either empty vector or Gli2 DNA construct and treated as ina. (c) LC3-II levels were detected by western blotting of total lysates from wild-type and Gli2−/− mice embryos (E12.5). For quantification, LC3-II levels from a total of five wild-type and five Gli2−/− embryos were normalized to actin, wild-type was set to 100. Graphs show mean values and error bars represent s.d. Statistical analysis were performed by two-tail Student’st-test **P<0.01. Pmph, purmorphamine. Figure 4: Hh regulation of autophagy is Gli2 dependent. ( a ) Wild-type Gli+/+ or Gli1−/−, Gli2−/− and Gli3−/− MEFs were treated with 100 mM trehalose alone or in combination with 10 μM of Pmph for 24 h, or left untreated. Total cell lysates were subjected to immunoblot with anti-LC3 and anti–actin antibodies. ( b ) Gli2−/− MEFs were transfected for 48 h with either empty vector or Gli2 DNA construct and treated as in a . ( c ) LC3-II levels were detected by western blotting of total lysates from wild-type and Gli2−/− mice embryos (E12.5). For quantification, LC3-II levels from a total of five wild-type and five Gli2−/− embryos were normalized to actin, wild-type was set to 100. Graphs show mean values and error bars represent s.d. Statistical analysis were performed by two-tail Student’s t -test ** P <0.01. Pmph, purmorphamine. Full size image To confirm these findings, we transfected Gli2-knockout MEFs with a Gli2 DNA construct and we made two important observations. First, overexpression of Gli2 was able to decrease LC3-II levels in Gli2−/− cells, confirming the role of Gli2 as a negative autophagy regulator, not only upon activation of the pathway with purmorphamine, but also in the absence of added stimuli. Second, confirming our previous data, Gli2−/− cells do not regulate autophagy upon purmorphamine treatment but this effect is rescued when Gli2 was exogenously expressed ( Fig. 4b ). Furthermore, whole lysates from Gli2−/− mouse embryos ( Fig. 4c ) showed a significant increase in the levels of endogenous LC3-II compared with their wild-type controls, suggesting that inactivation of Hh signalling as a consequence of Gli2 depletion leads to a constitutive activation of autophagy in samples of more biological relevance. Regulation of autophagy by Hh signalling in Drosophila To investigate the potential function of the Drosophila Hh pathway in autophagy, we first inactivated Hh signalling using a temperature-sensitive hedgehog allele, hh[ts2] . We followed autophagy by examining the formation of Lysotracker-positive vesicles in the larval fat body. This tissue is analogous to vertebrate liver/adipose tissue and has a robust, well-characterized autophagic response to starvation [32] . Fat bodies from wild-type control larvae remained essentially Lysotracker-negative at the 29 °C restrictive temperature ( Fig. 5a ), whereas incubation of hh[ts2] larvae at the restrictive temperature led to a marked induction of Lysotracker-positive punctae throughout the larval fat body ( Fig. 5b ). 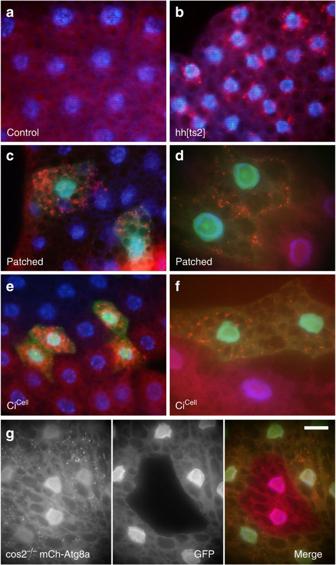Figure 5: Inactivation of Hedgehog signalling induces autophagy in theDrosophilalarval fat body. (a,b) Control (a) orhh[ts2](b) larvae were incubated at permissive temperature (18 °C) to the third instar stage, then cultured at non-permissive temperature (29 °C) in well-fed conditions for 24 h. Dissected fat body tissue was incubated in Lysotracker Red and DAPI and imaged unfixed. (c) Lysotracker Red-labelled fat body containing single-cell flipout clones (GFP positive) overexpressing patched. Fat body was dissected from well-fed larvae, incubated in Lysotracker Red/DAPI and imaged unfixed. (d) Confocal image of a GFP-positive patched-expressing clone, with mCherry-Atg8a expressed in all cells. Fat body was dissected from well-fed larvae and imaged after formaldehyde fixation. (e) GFP-marked flipout clones of CiCell-expressing cells. Fat body was dissected from well-fed larvae, incubated in Lysotracker Red/DAPI and imaged unfixed. (f) Confocal image of fixed mCherry-Atg8a expressing fat body containing a GFP-marked clone of CiCell-expressing cells. (g) Cells homozygous for the nullcostal2[2]allele (marked by lack of GFP) were generated by flp/FRT-mediated recombination in mCh-Atg8a expressing fat body. Larvae were starved 4 h before dissection and fixation. Scale bar represents 25 μm ina,b,cande, and 10 μm indandf. Genotypes: (a)y,w;(b)hh[ts2/ts2];(c)hs-flp; UAS-ptc/+; Act>CD2>GAL4 UAS-GFPnls/+;(d)hs-flp; UAS-ptc/+; r4:mCherry-Atg8a Act>CD2>GAL4 UAS-GFPnls/+;(e) hs-flp; UAS-CiCell/+; Act>CD2>GAL4 UAS-GFPnls/+;(f) hs-flp; UAS-CiCell/+; r4:mCherry-Atg8a Act>CD2>GAL4 UAS-GFPnls/+; (g) hs-flp; FRT42D cos2[2]/Cg-GAL4 UAS-mChAtg8a[2L] FRT42D UAS-GFPnls. Figure 5: Inactivation of Hedgehog signalling induces autophagy in the Drosophila larval fat body. ( a , b ) Control ( a ) or hh[ts2] ( b ) larvae were incubated at permissive temperature (18 °C) to the third instar stage, then cultured at non-permissive temperature (29 °C) in well-fed conditions for 24 h. Dissected fat body tissue was incubated in Lysotracker Red and DAPI and imaged unfixed. ( c ) Lysotracker Red-labelled fat body containing single-cell flipout clones (GFP positive) overexpressing patched. Fat body was dissected from well-fed larvae, incubated in Lysotracker Red/DAPI and imaged unfixed. ( d ) Confocal image of a GFP-positive patched-expressing clone, with mCherry-Atg8a expressed in all cells. Fat body was dissected from well-fed larvae and imaged after formaldehyde fixation. ( e ) GFP-marked flipout clones of Ci Cell -expressing cells. Fat body was dissected from well-fed larvae, incubated in Lysotracker Red/DAPI and imaged unfixed. ( f ) Confocal image of fixed mCherry-Atg8a expressing fat body containing a GFP-marked clone of Ci Cell -expressing cells. ( g ) Cells homozygous for the null costal2[2] allele (marked by lack of GFP) were generated by flp/FRT-mediated recombination in mCh-Atg8a expressing fat body. Larvae were starved 4 h before dissection and fixation. Scale bar represents 25 μm in a , b , c and e , and 10 μm in d and f . Genotypes: ( a ) y,w; ( b ) hh[ts2/ts2]; ( c ) hs-flp; UAS-ptc/+; Act>CD2>GAL4 UAS-GFPnls/+; ( d ) hs-flp; UAS-ptc/+; r4:mCherry-Atg8a Act>CD2>GAL4 UAS-GFPnls/+; ( e ) hs-flp; UAS-Ci Cell /+; Act>CD2>GAL4 UAS-GFPnls/+; ( f ) hs-flp; UAS-Ci Cell /+; r4:mCherry-Atg8a Act>CD2>GAL4 UAS-GFPnls/+ ; ( g ) hs-flp; FRT42D cos2[2]/Cg-GAL4 UAS-mChAtg8a[2L] FRT42D UAS-GFPnls. Full size image Accumulation of active lysosomes in response to inactivation of Hh could reflect either a direct role for Hh signalling in the fat body, or a non-autonomous response to reduced signalling in another organ(s). To distinguish between these possibilities, we inactivated the pathway within individual fat body cells through clonal overexpression of Ptch, using the flip-out Gal4-upstream activating sequence system [33] . This resulted in a cell autonomous induction of punctate Lysotracker staining exclusively in the Ptch-expressing cells ( Fig. 5c ). Patched overexpression also led to accumulation of vesicles marked with fluorescently labelled Atg8a, a Drosophila ortholog of mammalian LC3 and yeast Atg8 that localizes to autophagosomes and autolysosomes ( Fig. 5d ). Interestingly, the density of Ptch-induced mCherry-Atg8a punctae was skewed towards the cell periphery, in contrast to the more uniform distribution of these vesicles typically observed in response to starvation ( Supplementary Fig. S4A,B ). Consistent with the role of Gli2 in regulating autophagy in mammals, expression of a truncated, constitutively repressive form of the single fly ortholog of mammalian Gli proteins Ci, Ci Cell (ref. 34 ), resulted in a robust, cell autonomous induction of Lysotracker and mCherry-Atg8a labelled cytoplasmic punctae ( Fig. 5e ). Similar effects were observed when Ci expression was reduced by RNAi-mediated depletion ( Supplementary Fig. S4C ). Together, the induction of both autophagosomes and lysosomes in response to inactivation of Hh signalling are consistent with increased autophagic flux under these conditions. Whereas Hh inactivation led to a robust induction of autophagy, we found that activation of this pathway in fat body cells had milder effects. Induction of autophagy by starvation was not blocked by expression of an active, non-diffusible form of Hh nor by an uncleavable, active isoform of Ci (data not shown). Mutations in smoothened also had no effect on autophagy (data not shown). The effect of patched null mutations on autophagy was investigated in starved fat body cells by Lysotracker staining, which label autolysosomes, and by detecting endogenous levels of the selective autophagy substrate p62/Ref(2)P, which has been shown to accumulate in autophagy-defective cells. In both cases, ptc null cells were indistinguishable from surrounding wild-type cells ( Supplementary Fig. S5A–D ). In Drosophila , costal2 is part of the Hh signalling complex, where it interacts with Ci and is a negative regulator of Hh signalling. We found that cells mutant for costal2 showed a reduction in starvation-induced autophagosome production ( Fig. 5g ). This result suggests that the inhibitory effects of Hh signalling activation on autophagy may be mild compared with the robust induction of autophagy seen following starvation. Hh signalling regulates the autophagy modulator PERK In search for transcription targets of the Hh pathway that could constitute potential autophagy modulators, an exhaustive literature search extracted more than 2,000 unique genes that may be transcriptionally regulated by Hh pathway (see Supplementary Table S1 for references), which included a series of known autophagy genes ( Supplementary Table S2 ). Among these genes, we noted Bcl2 ( [35] ) and cFlip [36] , which have been reported to be specifically upregulated by Gli2, and both are known to inhibit autophagy [37] , [38] . However, Bcl2 and cFlip levels were not obviously altered in lysates from cells expressing Ptch1 or Ptch2 or after Ptch2 knockdown, relative to control cells ( Supplementary Fig. S6A ) and Bcl2 levels were also not changed in Gli2−/− embryos (data not shown). We next attempted a more direct strategy by analysing changes in the expression profile of 84 autophagy genes in response to Hh ligand using a PCR array approach ( Fig. 6a ). To our surprise, we did not detect any genes with significantly increased expression upon Hh treatment (we excluded those genes with very low expression, bottom-left part of the graph). However, of the 10 top candidates that had ~2-fold decreases in mRNA levels ( Fig. 6b ), two of them, PERK and GABARAPL1, had already been described as transcription targets of the Hh pathway ( Supplementary Table S2 ). We excluded ARSA, as this arylsulfatase has been related to lysosomal function, but no direct roles in autophagosome synthesis, such as we see with Hh modulation, have been reported. 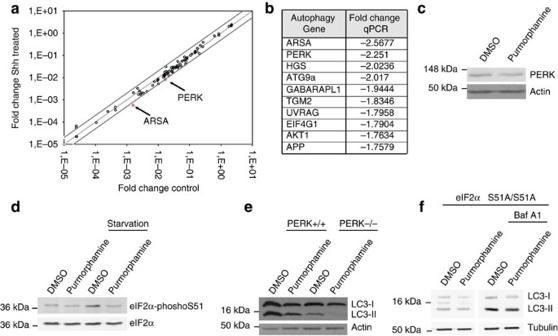Figure 6: Search of Hh transcriptional targets that regulate autophagy. (a) Graph representing fold change in mRNA levels in cells treated with Shh against untreated cells. Each circle represents an autophagy gene; those with largest fold-changes are indicated in red. The central line represents no changes in expression; above the central line, genes whose expression is increased: below, those with reduced levels. Grey lines indicate 2-fold increase or decrease. (b) Table showing the 10 genes with higher fold changes in expression and the values obtained. (c) Levels of PERK protein were assessed by western blotting in HeLa cells treated with 10 μM purmorphamine for 24 h. Actin was used as a protein loading control. (d) HeLa cells were treated with purmorphamine for 24 h and either left in rich media or in HBSS for the last 4 h. Levels of S51 phoshorylation and total levels of eIF2α were detected by western blotting using LI-COR infra-red imager. (e,f) Wild-type and PERK−/− (e) or eIF2α S51A/S51A MEFs (f) were treated with DMSO or 10 μM purmorphamine for 24 h and, where indicated, cells were treated with bafA1 for the last 4 h. LC3-II and actin or tubulin, as a loading control, were detected and a representative blot is shown. HBSS, Hank's balanced salt solution. Figure 6: Search of Hh transcriptional targets that regulate autophagy. ( a ) Graph representing fold change in mRNA levels in cells treated with Shh against untreated cells. Each circle represents an autophagy gene; those with largest fold-changes are indicated in red. The central line represents no changes in expression; above the central line, genes whose expression is increased: below, those with reduced levels. Grey lines indicate 2-fold increase or decrease. ( b ) Table showing the 10 genes with higher fold changes in expression and the values obtained. ( c ) Levels of PERK protein were assessed by western blotting in HeLa cells treated with 10 μM purmorphamine for 24 h. Actin was used as a protein loading control. ( d ) HeLa cells were treated with purmorphamine for 24 h and either left in rich media or in HBSS for the last 4 h. Levels of S51 phoshorylation and total levels of eIF2α were detected by western blotting using LI-COR infra-red imager. ( e , f ) Wild-type and PERK−/− ( e ) or eIF2α S51A/S51A MEFs ( f ) were treated with DMSO or 10 μM purmorphamine for 24 h and, where indicated, cells were treated with bafA1 for the last 4 h. LC3-II and actin or tubulin, as a loading control, were detected and a representative blot is shown. HBSS, Hank's balanced salt solution. Full size image GABARAPL1 belongs to the family of LC3 proteins and is also lipidated and associated with autophagic vesicles [39] . Treating Atg5-deficient MEFs with purmorphamine allows us to look at variations in the levels of this protein without the complication of protein lipidation. However, we were unable to detect any changes in levels of GABARAPL1 protein in these conditions ( Supplementary Fig. S6B ). PRK-like ER kinase (PERK or EIF2AK3) is an ER-resident protein responsible for the phosphorylation of eukaryotic initiation factor 2α (eIF2α), which inhibits protein translation in response to ER stress [40] . Hh pathway activation decreased PERK expression, as purmorphamine treatment reduced PERK protein levels ( Fig. 6c ), which was concomitant with a reduction in eIF2α phosphorylation at serine 51 both under basal conditions and following starvation ( Fig. 6d ). As growing evidence implicates PERK and eIF2α in autophagy regulation [41] , [42] , [43] ( Supplementary Fig. S6C ), we hypothesized that the PERK–EIF2α pathway was an effector of Hh-dependent autophagy. To further investigate the role of PERK in Hh signalling to autophagy, we used PERK-knockout MEFs and found that they still displayed a degree of autophagy inhibition in response to purmorphamine treatment ( Fig. 6e and supplementary Fig. S6D ). This result suggests that although PERK is a novel effector of the Hh pathway, additional mechanisms might be involved. Besides PERK, three other kinases phosphorylate EIF2α in mammalian cells: GCN2 in response to amino-acid starvation, PKR upon viral infection and HRI in haem deficiency. To establish whether these kinases provided the additional mechanisms by which Hh signalling controls autophagy, we investigated the ability of purmorphamine to reduce autophagy in MEFs where eIF2α cannot be phosphorylated [44] . In these cells, purmorphamine still reduced LC3-II levels ( Fig. 6f ), indicating that eIF2α phosphorylation is not the only signalling pathway involved in the control of autophagy by Hh. Our data indicate that Hh signalling regulates autophagy. These results have been validated in mammalian cells and Drosophila , and confirmed at different steps of the Hh pathway. In Drosophila , a single Ptch receptor responds to Hh molecules, whereas in mammalian cells Ptch1 and Ptch2 share this function. Although knockdown of Ptch1 did not inhibit autophagy in basal conditions, activation of the Hh pathway was not as efficient with Ptch1 compared with Ptch2 knockdown. Also, Ptch1 is a transcriptional target of the Hh pathway and its expression is expected to increase when the pathway is activated by Ptch1 siRNA treatment [12] . This feedback implies that Ptch1 siRNA may not be efficient enough to completely counteract its own transcriptional activation. Although more detailed experiments would be needed to rule out a differential contribution of these receptors, our data suggest that Shh modulates autophagy through Ptch1 and/or Ptch2. Gli transcription factors have distinct activator and repressor functions and their roles differ during embryonic development [28] , [29] . Although we cannot completely exclude a contribution of Gli1 and Gli3 to autophagy regulation, we confirmed that Gli2 is necessary for the inhibition of autophagy by Hh signalling. The increased LC3-II levels in Gli2-knockout embryos further confirmed our data in a biologically relevant context. These data do not explain the developmental defects in these mice but might suggest that some of their phenotypes could be secondary to autophagy dysregulation. However, almost certainly, factors other than autophagy inhibition will have major contributions to the developmental defect in these Gli2-knockout mice. Equally, we cannot exclude the possibility that other pathways that increase autophagy could be aberrantly activated in these embryos. Despite the effects of Gli2 and Ci on autophagy, the role of their upstream activator Smo was less clear-cut. This is not surprising, as it has been shown that Smo levels are not sufficient to stimulate the pathway, but an activation process is required, with Ptch influencing the transition to an active state of Smo in response to Shh [45] . In Drosophila , null mutations in Smo did not influence autophagy whereas Costal2 inhibition did, and it is therefore also possible that the Hh/Ptch complex and Ci may partially bypass Smo in Drosophila , consistent with the effects of this pathway on Costal2 localization to endomembranes [46] . Consequently, our data suggest that canonical and non-canonical Hh mechanisms might be involved in regulating autophagy, or that other factors might be necessary in Hh-mediated regulation of autophagy. Hh inhibition has been largely pursued as a therapeutic strategy for types of cancer resulting from a hyperactivation of the pathway, such as basal cell carcinomas or medulloblastoma [7] . Although the roles of autophagy in cancer are controversial and complex [47] , [48] , it is interesting to consider whether inhibition of autophagy by Hh would exacerbate or prevent the progression of these tumours when searching for pharmacological strategies. Cyclopamine, which binds and inhibits Smo [26] , is one of the best characterized Hh signalling inhibitors and it has been shown to be protective in Hh-related cancers [49] , [50] . As expected, cyclopamine caused LC3-II accumulation ( Supplementary Fig. S7A ). In the presence of bafA1, the increase was not as large as in non-treated cells ( Supplementary Fig. S7A ). This result was unexpected because bafA1 should exacerbate the changes on LC3-II if cyclopamine is triggering autophagosome synthesis, suggesting that cyclopamine might also affect autophagosome maturation. Consistent with an impairment in autophagosome degradation, cyclopamine and bafA1 both similarly reduced the number of acidic vesicles in mRFP-GFP-LC3 cells ( Supplementary Fig. S7B ). These data suggest that cyclopamine affects autophagosome degradation but that this effect is independent of Hh inhibition, as cyclopamine could increase LC3-II levels even in Gli2-null MEFs ( Supplementary Fig. S7C ). Our data suggest that cyclopamine has two opposite effects on autophagy. It increases autophagosome synthesis by inhibiting Smo activity, but it simultaneously impairs autophagosome maturation through an unknown mechanism that is independent of Gli2. Effects of cyclopamine independent of Smo inhibition have been reported in human breast cancer cell lines [51] and in zebrafish [52] , suggesting that this drug has additional molecular targets. In search of potential Hh transcriptional targets that could modulate autophagy, we identified PERK as the more consistent potential target and, in agreement with our observation, Eichberger et al . [53] previously reported that PERK is repressed upon Gli1 and Gli2 induction. This report also suggested that expression of Gli2 repressed a considerably larger number of genes than Gli1, an observation that may be of relevance when considering the more dominant effect of Gli2 on autophagy. Although Gli2 acts mainly as a transcriptional activator upon Hh activation, it can be proteolytically processed into a transcriptional repressor [54] , similar to the dual function of Ci in Drosophila. The autophagy inhibitory action of Gli2 can be explained by either a gain of repressor function towards some genes (such as PERK) in its active form, or by the fact that when activated it leads to increased expression of a second transcriptional repressor. It remains to be elucidated which of these mechanisms is in action in the case of PERK transcription. In response to unfolded proteins in the ER lumen, PERK is activated and phosphorylates eIF2α, increasing translation of the transcription factor ATF4 [40] . The exact mechanism by which eIF2α controls autophagy is unknown, eIF2α regulates Atg12 levels in the presence of expanded polyglutamines [41] and ATF4 has been suggested to increase transcription of Atg5 and LC3 (ref. 42 ). Indeed our PCR Array data show that levels of Atg5 upon Shh ligand are decreased to 0.8-fold compared with control cells. However, it is unlikely that this is the complete mechanism, as it has yet to be conclusively demonstrated that transcriptional induction of LC3 and Atg5 upregulate autophagy. It is also possible that PERK interacts more directly with other signalling pathways involved in autophagy regulation. As an example, the transcription factor Nrf2, known to be involved in autophagy regulation [55] , is phosphorylated by PERK independently of eIF2α in response to ER stress, promoting its import to the nucleus and activation of transcription [56] . In conclusion, these data not only provide insights into the connection between Hh and autophagy but also into the potential implications that Hh has in controlling protein homeostasis in physiological and disease conditions. Cell culture HeLa cells, wild-type Atg5+/+ and Atg5−/− MEFs (gift from N. Mizushima), wild-type Gli+/+, Gli1−/−, Gli2−/− and Gli3−/− MEFs (kindly provided by R. Lipinski) and PERK−/− MEFs (CRL-2976, ATCC), were grown in Dulbecco’s modified eagle medium supplemented with 10% FBS, 100 U ml −1 penicillin/streptomycin and 2 mM L -glutamine at 37 °C, 5% CO 2 . HeLa cells stably expressing mRFP-GFP-LC3 (ref. 57 ) were maintained in similar media supplemented with 600 μg ml −1 of G418. eIF2α A/A MEFs media was supplemented with non-essential amino acids and 2-mercaptoethanol. For starvation experiments cells were washed once with HBSS-containing calcium and magnesium and then incubated in this medium for 4 h. DNA constructs The 8xGli-luciferase and pcDNA3.1-HisB-Gli2 constructs [15] were kindly provided by H. Sasaki, pcI-Ptch1-1B and pcDNA3.1/HisB-Ptch2 (refs 58 , 59 ) by P. Zaphiropoulos; Smo-Myc 3 , SmoA1-Myc 3 and Smo-GFP constructs [26] by J. Chen and eIF2α by D. Ron (Addgene plasmid 21807). pcDNA3.1 empty vector was used as a control. The first exon of the huntingtin protein with 74 polyglutamines, tagged with EGFP or HA in N-terminal, EGFP-HttQ74 and HA-HttQ74, has been extensively characterized [16] . Gli2−/− mice embryo analysis Whole E12.5 and E13.5 wild-type and Gli2−/− mouse embryo lysates were kindly provided by A.L. Joyner. Embryos were lysed in RIPA buffer, resuspended in loading buffer and boiled before analysis by western blotting. Reagents Chemical compounds used in cell culture were N-Shh (10 μg ml −1 ; R&D Systems), bafA1 (400 nM, dimethylsulphoxide (DMSO; Millipore), purmorphamine (10 μM, DMSO; Santa Cruz), cyclopamine (10 μM, DMSO; Sigma), rapamycin (0.2 μg ml −1 , DMSO; Sigma) and trehalose (100 mM; Sigma). Autophagy assesment by automated Cellomics microscope HeLa cells stably expressing the mRFP-GFP-LC3 construct were fixed and stained with 4',6-diamidino-2-phenylindole (DAPI) and the analysis of the number of GFP and RFP-positive vesicles per cell was performed on a Thermo Scientific Cellomics ArrayScan HCS reader (40 × objective), using the Spot detector V3 Cellomics Bioapplication. Number of vesicles per cell was counted in one thousand cells per coverslip and the mean number of vesicles per cell was calculated by the ArrayScan software. Analysis was done on triplicate samples. HaloTag-p62 clearance assay for autophagy activity U2OS cell lines stably expressing HaloTag-p62 were generated. HaloTag-p62 plasmid was obtained from the Kazusa DNA Research Institute collection, the vector was linearized by digestion with Sca I and co-transfected with linear hygromycin marker (Clontech) into U2OS cells. Transfected cells were selected by culturing in the presence of hygromycin B. Following the establishment of a hygromycin B-resistant cell line, cells were labelled with diAcFam-conjugated HaloTag ligand (Promega) and single cells expressing HaloTag-p62 were sorted into individual wells of a 96-well plate by fluorescence-activated cell sorting. These cells were then cultured in the presence of 100 μg ml −1 hygromycin B to generate single-cell clones. To assay clearance of p62, cells were plated into 12-well plates and the following day they were labelled with HaloTag diAcFam fluorescent ligand (Promega) following the manufacturer’s instructions. After labelling, cells were treated with bafA1 (50 nM), rapamycin (200 nM), trehalose (100 mM), purmorphamine (10 μM) or DMSO as a control for 48 h total time (media was changed after 24 h). Cells were then collected as described for western blot samples above and run on SDS–polyacrylamide gel electrophoresis. Gels were scanned on a Typhoon 8600 variable mode imager. To allow for accurate quantification of total protein loading, gels were fixed and stained with Krypton Flourescent Protein Stain (Pierce) following the manufacturer’s instructions and fluorescence was measured on a Typhoon 8600 variable mode imager. Densitometric analysis of fluorescence levels was carried out using Image J software. Immunofluorescence and confocal microscopy Imaging was performed on a Zeiss Axiovert 200M microscope with an LSM 710 confocal atttachment, using a 63 × 1.4 numerical aperture Plan Apochromat oil-immersion lens. Autophagy expression profile PCR array The Human Autophagy RT2 Profiler PCR Array (SABiosciences, Frederick, MD) was used to study the expression profile of 84 autophagy-specific genes according to the manufacturer’s procedure. Briefly, total RNA was extracted from cells treated with Hh peptide or non-treated cells using Trizol (Invitrogen) and further purified using RNeasy mini kit with on-column DNAse digest (Qiagen), cDNA was then synthesized using an RT2 First strand kit (SABiosciences) and real-time PCR was performed using 7900HT fast real time PCR system (Applied Biosciences). Data were analysed with RT 2 profiler PCR array data analysis software version 3.5. Statisitical analysis Quantification of immunoblots was performed by densitometric analysis using the Image J software and normalized to loading control (actin or tubulin, as indicated). The P -values were determined by two-tail Student’s t -test in a triplicate experiment representative of at least three independent experiments. Statistical significancy of percentage of HttQ74 aggregates was determined by unconditional logistical regression analysis using the general log linear analysis option of SPSS Version 6.1 (SPSS, Chicago, IL, USA). Fat body and imaginal disc histology Larvae were cultured in plastic vials under non-crowded conditions in standard Drosophila cornmeal/molasses/agar media at 25 °C (fed conditions) or transferred to vials containing 20% sucrose for 4 h (starvation conditions). Heat shock-induced flippase/flippase recognition target (FRT)-mediated loss of function clones were induced at 0–6 h of embryogenesis (fat body clones) or 48 h by a 1-h heat shock at 37 °C and were marked by fat body-specific activation of upstream activating sequence-GFP lines on FRT-linked chromosomes. Gain-of-function (flip-out) clones were generated through spontaneous heat shock-induced flippase-dependent activation of Act>CD2>GAL4. Lysotracker staining was performed as described [32] , using fat body dissected from early third instar larvae (96 h) in 100 nM Lyso Tracker Red DND-99 (Invitrogen), 1 μg ml −1 DAPI (Sigma) in phosphate buffered saline (PBS). Stained fat body lobes were imaged in PBS on glass slides using a Zeiss Axioscope-2 microscope equipped with a Nikon DXM1200 digital camera (Melville, NY), using a × 40 Plan-Neofluar 0.75 NA objective lens and Nikon ACT-1 software. Samples for immunohistochemistry, GFP and mCherry visualization were fixed overnight at 4 °C in 3.7% formaldehyde/PBS, with Triton X-100 (0.1%)/BSA (1%)/PBS (PBT) used for post-fixation and antibody incubation washes. Larval carcasses were incubated overnight with primary antibodies diluted 1:1000 in PBT (rabbit anti-Ref(2)P, gift of T. Rusten) and overnight in Texas Red-labelled secondary antibodies (1:500, Jackson Immunolabs, West Grove, PA). Fat body and imaginal discs were mounted in Vectashield (Vector Laboratories, Burlingame, CA) and imaged with a Zeiss Axioplan-2 microscope (Thornwood, NY) equipped with a CARV spinning disk system and a Hamamatsu ORCA-ER digital camera (Bridgewater, NJ), using a × 63 Plan-Apochromat 1.4 NA objective lens and Axiovision software or an Axio Observer.Z1 microscope with LSM 710 confocal attachment. See Supplementary Information for extended Material and Methods. How to cite this article: Jimenez-Sanchez, M. et al . The Hedgehog signalling pathway regulates autophagy. Nat. Commun. 3:1200 doi: 10.1038/ncomms2212 (2012).